IKKα restoration via EZH2 suppression induces nasopharyngeal carcinoma differentiation Lack of cellular differentiation is a key feature of nasopharyngeal carcinoma (NPC), but it also presents as a unique opportunity for intervention by differentiation therapy. Here using RNA-seq profiling analysis and functional assays, we demonstrate that reduced IKKα expression is responsible for the undifferentiated phenotype of NPC. Conversely, overexpression of IKKα induces differentiation and reduces tumorigenicity of NPC cells without activating NF-κB signalling. Importantly, we describe a mechanism whereby EZH2 directs IKKα transcriptional repression via H3K27 histone methylation on the IKKα promoter. The differentiation agent, retinoic acid, increases IKKα expression by suppressing EZH2-mediated H3K27 histone methylation, resulting in enhanced differentiation of NPC cells. In agreement, an inverse correlation between IKKα (low) and EZH2 (high) expression is associated with a lack of differentiation in NPC patient samples. Collectively, these findings demonstrate a role for IKKα in NPC differentiation and reveal an epigenetic mechanism for IKKα regulation, unveiling a new avenue for differentiation therapy. Differentiation therapy holds great promise for cancer treatment and has yielded remarkable outcomes in certain type of cancers [1] , [2] , [3] , [4] , [5] , [6] , but the molecular mechanisms involved remain elusive. Nasopharyngeal carcinoma (NPC) is a distinctive type of head and neck cancer. More than 95% of NPCs are pathologically diagnosed as Type III undifferentiated carcinomas. Patients with this diagnosis have a much higher mortality rate than those diagnosed with well-differentiated Type I-keratinizing squamous cell carcinomas (SCCs) [7] . This clinical finding is consistent with the consensus view that lack of differentiation is an important hallmark of mammalian malignancy and progression [8] , [9] . This aspect of cancer biology presents a unique therapeutic opportunity. IκB kinase α (IKKα), also known as IKK1 and conserved helix-loop-helix ubiquitous kinase, is one of the two catalytic subunits of the IKK complex. Although IKKα is involved in nuclear factor-κB (NF-κB) activation, recent studies have shown this kinase also functions as a molecular switch that controls epidermal differentiation independent of its kinase activity in NF-κB signalling [10] , [11] , [12] , [13] , [14] . IKKα interacts with Smad2/3-containing transcription-activating complexes in a TGFβ-dependent manner and further induces the expression of Mad1, Mad2 and Ovol1 , all of which encode negative regulators of Myc during keratinocyte differentiation [15] . IKKα knockout mice display a hyperproliferative and undifferentiated epidermis, and IKKα-deficient keratinocytes fail to express terminal differentiation markers [16] . One recent study reported that IKKα reduction deregulated the expression of oncogenes, tumour suppressors and stem cell regulators in K5 + lung epithelial cells. The transition of IKKα low K5 + p63 hi cells to tumour cells played a pivotal role in spontaneous SCC development [17] . Conversely, overexpression of IKKα promotes epidermal differentiation, reduces keratinocyte proliferation and inhibits chemically induced SCC formation and progression. Notably, high-grade and poorly differentiated human SCCs display a loss of IKK α expression [18] . What is not known is the precise underlying molecular events that mediate IKKα repression. Epigenetic regulation plays a central role in gene regulation and differentiation. Polycomb group proteins form polycomb repressive complexes (PRCs) that are crucial epigenetic gene silencers during embryonic development and adult somatic cell differentiation [19] . PRC2 is originally identified as a silencer of Hox differentiation factors, a finding that has subsequently been expanded to dozens of other differentiation regulators. These include transcription factors of Gata, Sox, Fox, Pou and Pax families as well as components of the Wnt, TGF-β, Notch, FGF and retinoic acid signalling pathways [20] , [21] , [22] . The PRC2 consists of mammalian homologues of the Drosophila melanogaster proteins, including the enhancer of zeste (E (Z)), suppressor of zeste 12 (SU (Z) 12) and extra sex combs. The enhancer of zeste homologue 2 (EZH2) is the catalytically active component of the PRC2 complex. It preferentially represses target genes that initiate differentiation and restrain proliferation by inducing trimethylation of lysine 27 and lysine 9 of histone H3 (ref. 22 ). Indeed, genome-wide aberrant methylation has been observed in the majority of primary NPCs, indicating the importance of the epigenetic dysregulation during the process of NPC tumorigenesis [23] . However, the potential role of EZH2 in the regulation of cellular differentiation in NPC has not yet been elucidated. In the present study, we demonstrate that differentiation of NPC cells is impaired as a result of IKKα reduction. We show that the reduction in IKKα is caused by EZH2-mediated H3K27 histone methylation within the IKK α promoter. These new data establish an epigenetic mechanism by which EZH2 represses IKKα expression and impairs tumour cell differentiation. Downregulated IKKα leads to undifferentiated NPC status To identify the genes essential for NPC differentiation, we sequenced six RNA libraries from three paired NPC tumours (2T, 3T, 23T) as well as adjacent non-tumour (2N, 3N, 23N) tissues. Differential expression profiling of 3,163 deregulated genes was displayed as a heat map ( Fig. 1a ), where the genes were listed in descending order according to Baggerley’s test analysis. Thirteen genes (13/84) related to epithelial differentiation were downregulated in all three NPC patient samples compared with paired adjacent non-tumour tissues. Deregulation of seven candidate genes (7/13) was further confirmed by real-time quantitative PCR analysis ( Fig. 1b ), and they included ATF2, HES1, IKKα, KLF4, MAPK6, MAPK13 and NFATC4. We next explored the potential developmental role of these seven genes in the well-differentiated CNE1 cell line by gene silencing using siRNAs. As shown in the left panel of Fig. 1c , these siRNAs effectively downregulated mRNA expression of each of these seven genes. More importantly, western blot analysis showed that siRNA-mediated repression of either IKKα or NFATC4 significantly reduced expression of the epithelial cell differentiation markers involucrin and CK8 ( Fig. 1c right panel). In contrast, both IKKα and NFATC4 markedly increased expression of the squamous metaplasia dedifferentiation marker CK13. Subsequent experiments focused on IKKα because downregulation of IKKα mRNA level was also detected with five other pairs of primary NPC when compared with adjacent normal nasopharyngeal epithelium (2- to 22-fold, Fig. 1d left panel). Moreover, IKKα expression was also enriched in the normal nasopharyngeal epithelial cell line (NP69, >30-fold) as well as the well-differentiated NPC cell line (CNE1, >4-fold) compared with several poorly differentiated NPC cell lines (CNE2, SUNE1 and HONE1, Fig. 1d right panel). These data suggest that lack of IKKα expression is related to the undifferentiated state of NPC cells. 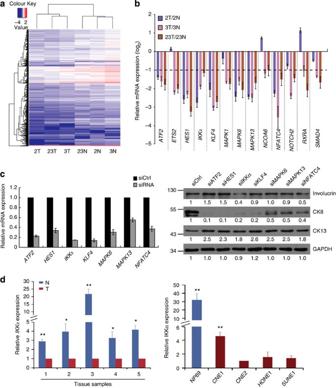Figure 1: IKKα downregulation is responsible for the undifferentiated phenotype of NPC. (a) An unbiased RNA-seq expression profiling heat map between normal nasopharyngeal tissues (2N, 3N, 23N) and NPC tissues (2T, 3T, 23T). High and low expression levels are indicated in red and blue, respectively. (b) The mRNA levels of 13 candidate genes in the three paired primary samples (2N, 2T, 3N, 3T, 23N and 23T) were verified with real-time PCR. (c) Repression of target genes was measured by real-time PCR (left panel). Involucrin, CK8 and CK13 levels in siRNAs transient-transfected CNE1 cells were analysed by western blot (right panel). (d) The mRNA level of IKKα in NPC specimens (left panel) and cell lines (right panel) was detected by real-time PCR. T: NPC tissues, N: paired normal nasopharyngeal tissues (n=3). NP69 is an immortalized normal human nasopharyngeal epithelial cell line. CNE1 is a well-differentiated NPC cell line, whereas CNE2, HONE1 and SUNE1 are poorly differentiated NPC cell lines. *P<0.05, **P<0.01 (two-tailed Student’st-tests). Error bars represent mean±s.d. Figure 1: IKKα downregulation is responsible for the undifferentiated phenotype of NPC. ( a ) An unbiased RNA-seq expression profiling heat map between normal nasopharyngeal tissues (2N, 3N, 23N) and NPC tissues (2T, 3T, 23T). High and low expression levels are indicated in red and blue, respectively. ( b ) The mRNA levels of 13 candidate genes in the three paired primary samples (2N, 2T, 3N, 3T, 23N and 23T) were verified with real-time PCR. ( c ) Repression of target genes was measured by real-time PCR (left panel). Involucrin, CK8 and CK13 levels in siRNAs transient-transfected CNE1 cells were analysed by western blot (right panel). ( d ) The mRNA level of IKKα in NPC specimens (left panel) and cell lines (right panel) was detected by real-time PCR. T: NPC tissues, N: paired normal nasopharyngeal tissues ( n =3). NP69 is an immortalized normal human nasopharyngeal epithelial cell line. CNE1 is a well-differentiated NPC cell line, whereas CNE2, HONE1 and SUNE1 are poorly differentiated NPC cell lines. * P <0.05, ** P <0.01 (two-tailed Student’s t -tests). Error bars represent mean±s.d. Full size image IKKα induces differentiation and decreases tumorigenicity To explore whether overexpression of IKKα inhibits proliferation of NPC cells and leads to their differentiation, we ectopically introduced either a control vector or wild-type IKKα in CNE2 cells. Forced expression of IKKα in poorly differentiated CNE2 cells led to marked morphologic changes that were comparable to well-differentiated NP69 or CNE1 cells. These changes were histologically characterized as a slender and fusiform phenotype ( Fig. 2a and Supplementary Fig. 1 ). Moreover, expression of involucrin and CK8 was increased, whereas CK13 expression was reduced ( Fig. 2b ). Similar results with forced expression of IKKα were observed in two other poorly differentiated NPC cell lines (HONE1 and SUNE1, Supplementary Fig. 2a ). In addition, CNE2-IKKα cells exhibited the downregulation of vimentin and upregulation of E-cadherin ( Fig. 2b ), indicative of NPC cell differentiation. Both cell number and colony formation assays showed that cell growth was significantly suppressed following overexpression of IKKα in CNE2 cells ( Fig. 2c,d ). In addition, overexpression of IKKα in CNE2 cells increased the G1 population, reduced cyclin D1 and cyclin E expression ( Supplementary Fig. 2b,c ), decreased the ratio of Ki67-positive cells and increased the proportion of senescence-associated (SA) β-gal-positive cells ( Fig. 2e,f ). Furthermore, overexpression of IKKα in CNE2 cells did not reduce the IκBα expression ( Fig. 2g , upper left panel), which inhibited NF-κB activity. Forced expression of IKKα also did not induce p65 nuclear translocation ( Fig. 2g , lower panel) and NF-κB target gene IL6 , IL8 transcription ( Fig. 2g , upper right panel). 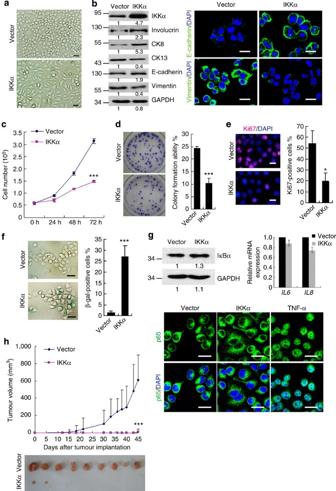Figure 2: Overexpression of IKKα induces differentiationin vitroand decreases tumorigenicityin vivo. (a) Phase contrast images of CNE2 cells expressing either control vector (pBabe) or pBabe-IKKα. (b) Western blot and immunofluorescence analysis with indicated antibodies in control (vector) and IKKα-overexpressed CNE2 cells. (c–f) IKKα-overexpressed and control (vector) CNE2 cells were subjected to determining the number of cells (n=3), ***P<0.001, two-tailed Student’st-tests (c), colony formation (n=3), ***P<0.001, two-tailed Student’st-tests (d), immunofluorescence staining of Ki67 (n=3), *P<0.05, two-tailed Student’st-tests (e) and SA-β-Gal staining (n=5), ***P<0.001, two-tailed Student’st-tests (f). (g) IKKα-overexpressed and control (vector) CNE2 cells were subjected to western blot, immunofluorescence staining of p65 and real-time PCR analysis. TNF-α was used as a positive control. (h) IKKα-overexpressed and control (vector) CNE2 cells (3 × 105cells per mouse) were injected into nude mice subcutaneously, and tumour volume was determined (n=9), ***P<0.001, two-tailed Student’st-tests. Scale bars, 50 μm (a,f); 25 μm (b,eandg). Error bars represent mean±s.d. Figure 2: Overexpression of IKKα induces differentiation in vitro and decreases tumorigenicity in vivo . ( a ) Phase contrast images of CNE2 cells expressing either control vector (pBabe) or pBabe-IKKα. ( b ) Western blot and immunofluorescence analysis with indicated antibodies in control (vector) and IKKα-overexpressed CNE2 cells. ( c – f ) IKKα-overexpressed and control (vector) CNE2 cells were subjected to determining the number of cells ( n =3), *** P <0.001, two-tailed Student’s t -tests ( c ), colony formation ( n =3), *** P <0.001, two-tailed Student’s t -tests ( d ), immunofluorescence staining of Ki67 ( n =3), * P <0.05, two-tailed Student’s t -tests ( e ) and SA-β-Gal staining ( n =5), *** P <0.001, two-tailed Student’s t -tests ( f ). ( g ) IKKα-overexpressed and control (vector) CNE2 cells were subjected to western blot, immunofluorescence staining of p65 and real-time PCR analysis. TNF-α was used as a positive control. ( h ) IKKα-overexpressed and control (vector) CNE2 cells (3 × 10 5 cells per mouse) were injected into nude mice subcutaneously, and tumour volume was determined ( n =9), *** P <0.001, two-tailed Student’s t -tests. Scale bars, 50 μm ( a , f ); 25 μm ( b , e and g ). Error bars represent mean±s.d. Full size image Given the phenotypic and functional changes we observed in CNE2 cells that overexpress IKKα cells in vitro , we next tested whether IKKα overexpression affected tumorigenicity in vivo by using a xenograft tumour model. As shown in Fig. 2h , distinct tumour masses were detected as early as 11 days in mice injected subcutaneously with CNE2-vector cells. In contrast, tumour masses could not be detected in mice injected with CNE2-IKKα even 40 days later ( Supplementary Table 1 ). Similarly, well-differentiated CNE1 cells had a markedly lower tumorigenic activity compared with poorly differentiated CNE2 cells ( Supplementary Table 1 ). In addition, the mouse tumours were examined with cell differentiation markers by immunohistochemical analysis. The tumours of mice injected with CNE2-IKKα cells showed markedly higher staining of IKKα, CK8 and involurcin compared with those injected with CNE2-vector control cells ( Supplementary Fig. 3 ). Taken together, these results suggest that IKKα induces differentiation and reduces tumorigenicity of NPC cells, which are not mediated through NF-κB signalling activation. IKKα is repressed by EZH2-mediated promoter H3 methylation To elucidate the mechanism that is responsible for the downregulation of IKKα in NPC, we examined the promoter region of IKK α and identified consensus polycomb response elements [24] ( Fig. 3a ). This finding raised the possibility that PRC2 might be involved in the repression of IKK α and led us to examine the expression and activity of PRC2 in NPC. We found high levels of the PRC2 component EZH2 as well as H3K27me3 modification in NPC compared with normal cells. Specifically, both EZH2 and H3K27me3 were highly elevated in the poorly differentiated CNE2, HONE1 and SUNE1 NPC cell lines compared with the normal nasopharyngeal epithelial cell line NP69 as well as well-differentiated NPC cells CNE1 ( Fig. 3b ). 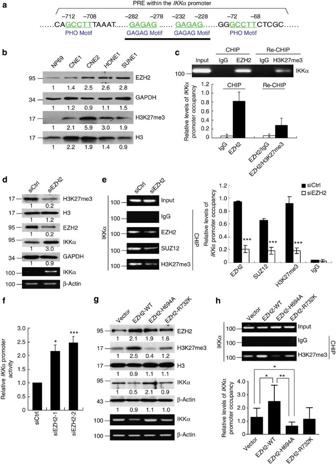Figure 3: IKKα is repressed by EZH2-mediated H3K27 histone methylation within theIKKα promoter. (a) Illustration of Polycomb response element (PRE) within theIKKα promoter. The sequence alignment of PRE within theIKKα promoter is shown (green letter: core DNA motifs of PRE, black bar: region amplified in CHIP-PCR). (b) Expressions of EZH2 and H3K27me3 in NPC cell lines were measured by western blot analysis. (c) Products of CHIP using an EZH2 antibody and Re-CHIP using an H3K27me3 antibody were subjected to PCR and real-time PCR in CNE2 cells. Data in the bottom panel are expressed as the fold of enrichment relative to the original input DNA. The ‘relative levels ofIKKα promoter occupancy’ were examined by real-time PCR and calculated using ΔCt value. (d,e) CNE2 cells were transfected with siEZH2 for 24 h and subjected to western blot (d, upper), RT–PCR (d, lower) and CHIP assay (n=3), ***P<0.001, two-tailed Student’st-tests (e). (f) CNE2 cells treated with siEZH2 for 24 h and subjected to dual-luciferase reporter assays. Data are shown as relativeIKKα promoter activity (n=3), *P<0.05, ***P<0.001, two-tailed Student’st-tests. (g,h) CNE2 cells expressing vector (pBabe), pBabe-EZH2-wild-type (EZH2-WT), pBabe-EZH2-H694A (EZH2-H694A) or pBabe-EZH2-R732K (EZH2-R732K) were analysed by western blot (g, upper), RT–PCR (g, lower) and CHIP with the indicated antibodies (n=7), *P<0.05, **P<0.01, two-tailed Student’st-tests (h). The ‘relative levels ofIKKα promoter occupancy’ were examined by real-time PCR and calculated using ΔCt value. Error bars represent mean±s.d. Figure 3: IKKα is repressed by EZH2-mediated H3K27 histone methylation within the IKK α promoter. ( a ) Illustration of Polycomb response element (PRE) within the IKK α promoter. The sequence alignment of PRE within the IKK α promoter is shown (green letter: core DNA motifs of PRE, black bar: region amplified in CHIP-PCR). ( b ) Expressions of EZH2 and H3K27me3 in NPC cell lines were measured by western blot analysis. ( c ) Products of CHIP using an EZH2 antibody and Re-CHIP using an H3K27me3 antibody were subjected to PCR and real-time PCR in CNE2 cells. Data in the bottom panel are expressed as the fold of enrichment relative to the original input DNA. The ‘relative levels of IKK α promoter occupancy’ were examined by real-time PCR and calculated using ΔCt value. ( d , e ) CNE2 cells were transfected with siEZH2 for 24 h and subjected to western blot ( d , upper), RT–PCR (d, lower) and CHIP assay ( n =3), *** P <0.001, two-tailed Student’s t -tests ( e ). ( f ) CNE2 cells treated with siEZH2 for 24 h and subjected to dual-luciferase reporter assays. Data are shown as relative IKK α promoter activity ( n =3), * P <0.05, *** P <0.001, two-tailed Student’s t -tests. ( g , h ) CNE2 cells expressing vector (pBabe), pBabe-EZH2-wild-type (EZH2-WT), pBabe-EZH2-H694A (EZH2-H694A) or pBabe-EZH2-R732K (EZH2-R732K) were analysed by western blot ( g , upper), RT–PCR ( g , lower) and CHIP with the indicated antibodies ( n =7), * P <0.05, ** P <0.01, two-tailed Student’s t -tests ( h ). The ‘relative levels of IKK α promoter occupancy’ were examined by real-time PCR and calculated using ΔCt value. Error bars represent mean±s.d. Full size image Next, we performed chromatin immunoprecipitation (CHIP) analysis to investigate whether EZH2 was associated with the IKK α locus. As shown in Fig. 3c , EZH2 bound to the GAGAG motif within the IKK α promoter where EZH2 and H3K27me3 were co-occupied, as revealed by CHIP and Re-CHIP assays. Then, by using siRNA to knock down EZH2, we found that H3K27me3 was reduced at the same time that both mRNA and protein expressions of IKKα were increased ( Fig. 3d ). In addition, the PRC2 complex proteins EZH2 and SUZ12, as well as H3K27me3, bound the IKK α promoter DNA much less efficiently in EZH2 siRNA-treated CNE2 cells compared with si-control cells ( Fig. 3e ). A dual-luciferase reporter assay established that transcriptional activity of IKK α increased significantly in siEZH2-treated CNE2 cells compared with control cells ( Fig. 3f ). Moreover, we transiently transfected either wild type (WT) or mutants (H694A, a SET domain mutant, and R732K, a C-terminus mutant related to retain the ability to methylate histone H3 [25] ) EZH2 cDNA in CNE2 cells. RT-PCR and western blot assays showed that IKKα expression was reduced in EZH2-WT cells compared with empty vector-transfected cells. In contrast, overexpression of the methyl-transferase mutant EZH2-H694A increased IKKα expression while reducing H3K27me3 levels compared with EZH2-WT and vector control ( Fig. 3g ). Consistently, CHIP assays showed that EZH2-WT increased, but EZH2-H694A mutant reduced, H3K27 histone methylation within the IKK α promoter when compared with vector control ( Fig. 3h ). EZH2-R732K mutant, which retained the histone methyl-transferase (HMT) activity, showed a slight non-significant decrease in IKKα expression compared with vector control ( Fig. 3g ). CHIP assays showed that the EZH2-R732K mutant retained the H3K27 methylation within the IKK α promoter comparable to vector control, but less efficient than that in EZH2-WT-expressing CNE2 cells ( Fig. 3h ). Collectively, these data provide evidence that H3K27 histone methylation mediated by EZH2, which requires the intact SET domain, is involved in silencing IKK α transcription. Recent studies strongly suggest that the establishment of the basic DNA methylation profile might be mediated through histone modification [26] . We thus analysed the methylation status of IKK α promoter by methylation-specific PCR (MSP). The CpG islands of IKK α gene were heavily methylated in NPC cell lines and samples compared with those in the non-cancer nasopharyngeal cell line and tissues ( Supplementary Fig. 4a,b ). To explore whether EZH2 is correlated with the DNA methylation of IKK α promoter, we performed the MSP assay in CNE2 cells silenced by EZH2 siRNA. Results showed that the methylated (M) IKK α promoter was reduced, whereas the unmethylated (U) promoter was increased in siEZH2-treated CNE2 cells ( Supplementary Fig. 4c ). These results suggested that EZH2-mediated histone methylation may contribute to DNA methylation in the IKK α promoter. EZH2 modulates differentiation and tumorigenicity of NPC These new findings suggested that silencing EZH2 might induce differentiation in NPC. To test this notion, we used siRNAs to suppress endogenous EZH2 in CNE2, HONE1 and SUNE1 cells. The results showed that silencing of EZH2 caused an increase in levels of IKKα, involucrin and CK8 and decrease of CK13 ( Fig. 4a and Supplementary Fig. 5 ). Suppression of EZH2 in CNE2 cells also led to increased E-cadherin and reduced vimentin expression ( Fig. 4a ), as well as morphological changes in CNE2 cells ( Fig. 4b ), similar to IKKα-induced NPC cell differentiation. To further test our hypothesis, we then stably expressed EZH2-shRNA in CNE2 cells (referred to as shEZH2 cells). Compared with CNE2 cells expressing a control shRNA, expression of EZH2 protein was markedly decreased in shEZH2 CNE2 cells ( Fig. 4c ). As expected, suppression of EZH2 markedly reduced proliferation of CNE2 cells ( Fig. 4d ). In addition, silencing of EZH2 in CNE2 cells caused a significant reduction in colony number ( Fig. 4e ). Finally, we subcutaneously injected CNE2 cells with either EZH2-shRNA or control shRNA into nude mice and evaluated tumour growth. In contrast to control CNE2 cells, which formed large tumours, shEZH2 CNE2 cells displayed greatly reduced tumour growth ( Fig. 4f ). In addition, immunohistochemical analysis revealed increased levels of IKKα, CK8, involucrin and E-cadherin with decreased vimentin staining in tumours of mice injected with shEZH2 CNE2 cells, compared with those injected with control cells ( Fig. 4g ). 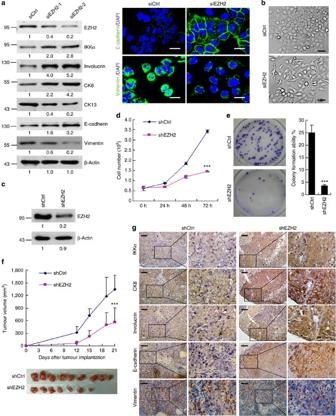Figure 4: Suppression of EZH2 in CNE2 cells induces differentiationin vitroand decreases tumorigenicityin vivo. (a) Expression of indicated proteins was analysed by western blot and immunofluorescence in siEZH2-treated CNE2 cells. (b) Morphology of siEZH2-treated CNE2 cells is shown by phase contrast photomicrographs. Scale bars, 50 μm. (c) Western blot assays showed that EZH2 expression is suppressed in shEZH2 CNE2 cells. (d,e) Proliferation of shEZH2 or sh-control CNE2 cells was analysed using both cell number (n=3), ***P<0.001, two-tailed Student’st-tests (d), colony formation assays (n=3), ***P<0.001, two-tailed Student’st-tests (e). (f) Mice were injected with shEZH2 or sh-control CNE2 cells subcutaneously (1 × 106cells per mouse). Tumour volume was determined as described in Methods (n=7–9), ***P<0.001, two-tailed Student’st-tests. (g) Immunohistochemical analysis of tumours from mice injected with CNE2-shEZH2 cells or control cells with IKKα, CK8, involucrin, E-cadherin and vimentin antibodies. Representative immunohistochemical images are shown. Scale bars, 25 μm (a); 50 μm (b), 100 μm (g). Error bars represent mean±s.d. Figure 4: Suppression of EZH2 in CNE2 cells induces differentiation in vitro and decreases tumorigenicity in vivo . ( a ) Expression of indicated proteins was analysed by western blot and immunofluorescence in siEZH2-treated CNE2 cells. ( b ) Morphology of siEZH2-treated CNE2 cells is shown by phase contrast photomicrographs. Scale bars, 50 μm. ( c ) Western blot assays showed that EZH2 expression is suppressed in shEZH2 CNE2 cells. ( d , e ) Proliferation of shEZH2 or sh-control CNE2 cells was analysed using both cell number ( n =3), *** P <0.001, two-tailed Student’s t -tests ( d ), colony formation assays ( n =3), *** P <0.001, two-tailed Student’s t -tests ( e ). ( f ) Mice were injected with shEZH2 or sh-control CNE2 cells subcutaneously (1 × 10 6 cells per mouse). Tumour volume was determined as described in Methods ( n =7–9), *** P <0.001, two-tailed Student’s t -tests. ( g ) Immunohistochemical analysis of tumours from mice injected with CNE2-shEZH2 cells or control cells with IKKα, CK8, involucrin, E-cadherin and vimentin antibodies. Representative immunohistochemical images are shown. Scale bars, 25 μm ( a ); 50 μm ( b ), 100 μm ( g ). Error bars represent mean±s.d. Full size image Derepression of IKKα by retinoic acid depends on EZH2 inhibition Retinoic acid (RA) is currently in use or being evaluated for several human cancers as a differentiation agent. Here we tested the hypothesis that differentiation therapy with RA would regulate pathways upstream of IKKα. As expected, we found that RA increased IKKα mRNA and protein levels in a dose-dependent manner ( Fig. 5a ). More importantly, RA decreased both EZH2 and H3K27me3 expression. CHIP analysis then revealed that binding of EZH2 and SUZ12 with the endogenous IKK α promoter region was significantly reduced in RA-treated CNE2 cells ( Fig. 5b ). Consistently, in the presence of RA, H3K27 histone methylation was also decreased within the IKK α promoter. Finally, by using a dual-luciferase reporter assay, we found that RA increased transcriptional activity of IKK α in CNE2 cells ( Fig. 5c ). 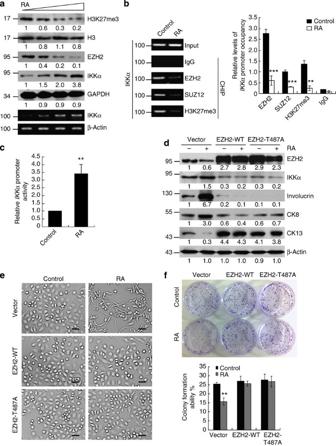Figure 5: Derepression of IKKα by RA depends on EZH2 inhibition. (a) CNE2 cells were treated with increasing doses (0, 10, 20 and 30 μM) of RA for 48 h and subjected to western blot (up panel) and RT-PCR analysis (lower panel). (b,c) CNE2 cells were incubated with RA (30 μM) for 48 h and subjected to CHIP (n=3), **P<0.01, ***P<0.001, two-tailed Student’st-tests (b), dual-luciferase reporter assays (n=3), **P<0.01, two-tailed Student’st-tests (c). (d–f) CNE2 cells expressing pCDNA3.1-EZH2 (WT or T487A) or vector (pCDNA3.1) were cultured with RA (30 μM) or control (DMSO) for 48 h and subjected to western blot analysis (d), phase contrast imaging (e), colony formation assay (n=3), **P<0.01, two-tailed Student’st-tests (f). Error bars represent mean±s.d. Scale bars, 50 μm (e). Figure 5: Derepression of IKKα by RA depends on EZH2 inhibition. ( a ) CNE2 cells were treated with increasing doses (0, 10, 20 and 30 μM) of RA for 48 h and subjected to western blot (up panel) and RT-PCR analysis (lower panel). ( b , c ) CNE2 cells were incubated with RA (30 μM) for 48 h and subjected to CHIP ( n =3), ** P <0.01, *** P <0.001, two-tailed Student’s t -tests ( b ), dual-luciferase reporter assays ( n =3), ** P <0.01, two-tailed Student’s t -tests ( c ). ( d – f ) CNE2 cells expressing pCDNA3.1-EZH2 (WT or T487A) or vector (pCDNA3.1) were cultured with RA (30 μM) or control (DMSO) for 48 h and subjected to western blot analysis ( d ), phase contrast imaging ( e ), colony formation assay ( n =3), ** P <0.01, two-tailed Student’s t -tests ( f ). Error bars represent mean±s.d. Scale bars, 50 μm ( e ). Full size image To investigate whether downregulation of EZH2 by RA is essential for IKKα expression and differentiation, we then overexpressed EZH2 (WT and T487A mutant) in CNE2 cells [27] , [28] . Consistent with this hypothesis, western blot analysis showed that RA was unable to enhance IKKα, involucrin or CK8 expression in both EZH2-WT- and -T487A-expressing cells ( Fig. 5d ). In contrast, RA increased IKKα, involucrin and CK8 expression in the control vector-expressing cells. In addition, RA-induced repression of CK13 in vector cells was abrogated in EZH2-WT and -T487A cells. Furthermore, in response to RA, slender and fusiform morphological changes were observed in control cells but not in EZH2-WT- or -T487A-expressing cells ( Fig. 5e ). Colony formation assays showed that proliferation of control cells was severely suppressed in the presence of RA. In contrast, there was no significant reduction in cell proliferation in RA-treated EZH2-WT- and -T487A-expressing cells ( Fig. 5f ). These results establish that RA restores IKKα expression by reducing EZH2-mediated H3K27 methylation in NPC cells. RA promotes NPC differentiation by inducing IKKα expression Next, we explored the possibility that RA would induce differentiation in NPC cells. As expected, western blot showed that RA increased IKKα protein in CNE2, HONE1 and SUNE1 cells ( Fig. 6a and Supplementary Fig. 6a ). These three poorly differentiated NPC cell lines incubated with RA displayed further induction of differentiation, as determined by increased levels of involucrin and CK8, and reduced CK13 expression. In addition, RA treatment also increased E-cadherin and reduced vimentin in CNE2 cells, as shown in the analysis by western blot and immunofluorescence staining ( Fig. 6a ). These changes were similar to those observed in CNE2-IKKα cells. Moreover, treatment with RA caused morphological changes indicative of differentiation, suppressed proliferation, colony formation and the number of Ki67-positive cells, and increased the proportion of SA β-gal-positive CNE2 cells ( Fig. 6b–d , Supplementary Fig. 6b,c ). 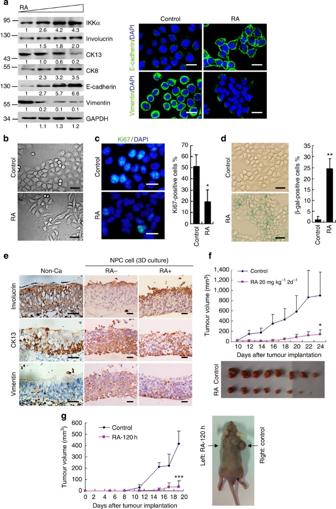Figure 6: RA promotes differentiation in poorly differentiated NPC cells by inducing IKKα expression. (a) CNE2 cells were treated with RA in increasing doses (0, 10, 20 and 30 μM) for 48 h and subjected to western blot and immunofluorescence analysis. (b) Morphology of RA treated (30 μM–48 h) or control (DMSO) CNE2 cells are shown by phase contrast photomicrographs. (c,d) CNE2 cells were treated with RA (30 μM) or control (DMSO) and subjected to immunofluorescence staining for Ki67 (n=3), *P<0.05, two-tailed Student’st-tests (c), SA-β-Gal staining (n=3), **P<0.01, two-tailed Student’st-tests (d). (e) Immunohistochemistry of involucrin, vimentin and CK13 in air–liquid interface 3D cultured CNE2 cells (control (DMSO): middle panel, RA (20 μM): right panel) and non-cancer specimens (left panel). (f) Mice were injected with CNE2 cells subcutaneously (1 × 106cells per mouse). At 10 days following injection, mice were treated with RA (20 mg kg−1(2d)−1, i.g.) or water (control). Tumour volumes were calculated as described in the Methods (n=8), *P<0.05, two-tailed Student’st-tests. (g) CNE2 cells were incubated with RA (30 μM) or control (DMSO) for 120 h and injected subcutaneously (1 × 106cells per mouse,n=5). Tumour volumes were determined as described in the Methods (n=5), ***P<0.001, two-tailed Student’st-tests. Scale bars, 25 μm (a,c); 50 μm(b,d,e). Error bars represent mean±s.d. Figure 6: RA promotes differentiation in poorly differentiated NPC cells by inducing IKKα expression. ( a ) CNE2 cells were treated with RA in increasing doses (0, 10, 20 and 30 μM) for 48 h and subjected to western blot and immunofluorescence analysis. ( b ) Morphology of RA treated (30 μM–48 h) or control (DMSO) CNE2 cells are shown by phase contrast photomicrographs. ( c , d ) CNE2 cells were treated with RA (30 μM) or control (DMSO) and subjected to immunofluorescence staining for Ki67 ( n =3), * P <0.05, two-tailed Student’s t -tests ( c ), SA-β-Gal staining ( n =3), ** P <0.01, two-tailed Student’s t -tests ( d ). ( e ) Immunohistochemistry of involucrin, vimentin and CK13 in air–liquid interface 3D cultured CNE2 cells (control (DMSO): middle panel, RA (20 μM): right panel) and non-cancer specimens (left panel). ( f ) Mice were injected with CNE2 cells subcutaneously (1 × 10 6 cells per mouse). At 10 days following injection, mice were treated with RA (20 mg kg −1 (2d) −1 , i.g.) or water (control). Tumour volumes were calculated as described in the Methods ( n =8), * P <0.05, two-tailed Student’s t -tests. ( g ) CNE2 cells were incubated with RA (30 μM) or control (DMSO) for 120 h and injected subcutaneously (1 × 10 6 cells per mouse, n =5). Tumour volumes were determined as described in the Methods ( n =5), *** P <0.001, two-tailed Student’s t -tests. Scale bars, 25 μm ( a , c ); 50 μm( b , d , e ). Error bars represent mean±s.d. Full size image To further characterize RA-induced differentiation, we performed an air–liquid interface three-dimensional (3D) culture assay ( Fig. 6e ). CNE2 cells formed a multi-layered tissue when cultured at an air–liquid interface, as described previously [29] . Immunohistochemical staining showed that the supra basal layer cells expressed higher levels of involucrin (apical marker) in the RA-treated group ( Fig. 6e , right panel) as compared with the DMSO-treated control group ( Fig. 6e , middle panel). Moreover, in the DMSO control tissue, the basal markers CK13 and vimentin were diffusely expressed throughout all cell layers. In contrast, CK13 and vimentin were mainly restricted to the basal layer in RA-treated tissue, which was similar to that observed in clinical non-cancer nasopharyngeal specimens ( Fig. 6e , left panel). To determine the effects of RA on tumorigenicity in vivo , we established subcutaneous flank xenograft tumours using CNE2, HONE1 and SUNE1 cells in nude mice. As shown in Fig. 6f and Supplementary Fig. 7a,b , RA treatment (i.g. 20 mg kg −1 per 2 days) resulted in a significant inhibition of tumour growth compared with control mice as indicated by decreased sizes of tumours ( n =5–8). In addition, CNE2 and SUNE1 cells pretreated with RA for 4 to 5 days showed significantly reduced tumorigenic capacity than control cells ( Fig. 6g and Supplementary Fig. 7c ). Immunohistochemistry revealed that treatment with RA resulted in induction of IKKα, CK8 and involucrin levels in tumour cells compared with control vehicle treatment ( Supplementary Fig. 7d ). To determine whether IKKα is required for RA-induced differentiation, we knocked down IKKα expression using siRNA before RA treatment in CNE2 cells. These experiments showed that RA increased expression of both involucrin and CK8 in control cells treated with a scrambled siRNA (si-control, Supplementary Fig. 8a ). However, induction of involucrin and CK8 was significantly inhibited in cells transfected with siIKKα. In addition, RA-induced repression of CK13 in si-control cells was abrogated in siIKKα cells. Moreover, we observed differentiation-associated morphological changes in si-control cells in response to RA, but not in RA-treated siIKKα cells ( Supplementary Fig. 8b ). In the presence of RA, the colony-forming ability of si-control cells was severely inhibited. In contrast, there was no significant difference in growth of RA-treated IKKα repression cells ( Supplementary Fig. 8c ). Low IKKα and high EZH2 correlate with undifferentiated NPC Collectively, all of these new data suggest that EZH2-mediated repression of IKKα expression contributes to both tumorigenesis and differentiation blockage in NPC. We therefore examined the expression of EZH2 in the primary human NPC samples and found that EZH2 was significantly higher in tumour samples compared with the paired adjacent normal nasopharyngeal epithelium ( Supplementary Fig. 9 ). Next, we used immunohistochemistry to determine expression of IKKα and EZH2 in primary human NPC and non-cancer nasopharyngeal samples. Clinical features of the patients are summarized in Supplementary Table 2 . The best cutoff points for parameters were determined by receiver operating characteristic curve analysis. A total of nine non-cancer nasopharyngeal mucositis and 87 NPC samples were evaluated. A significant portion of non-cancer nasopharyngeal samples (6/9, 66.7%) and differentiated NPC specimens (9/13, 69.2%) showed strong IKKα staining, but only a minority (26/74, 35.1%) of undifferentiated NPC samples displayed high IKKα staining ( Fig. 7a and Table 1 ). In addition, all non-cancer specimens showed EZH2-negative staining and only a few (3/13, 23.1%) of pathologically differentiated NPC specimens displayed EZH2-positive staining. In contrast, EZH2 was significantly elevated in a majority (63/74, 85.1%) of undifferentiated NPC specimens. Analysis by the Fisher's exact test showed that IKKα negatively and EZH2 positively correlated with undifferentiated status in NPC tissues ( Table 1 ). Furthermore, the median score of IKKα expression in undifferentiated NPC specimens was markedly lower compared with the differentiated NPC and non-cancer tissues, whereas EZH2 expression had the opposite tendency ( Fig. 7b ). Finally, we detected high EZH2 expression in 42 of 55 (76.4%) specimens with low IKKα expression, indicating a significant negative correlation between IKKα and EZH2 expression ( Table 2 ). 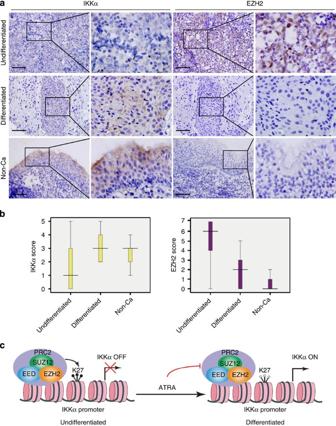Figure 7: Low IKKα and high EZH2 correlate with undifferentiated status in NPC tissues. (a) Human primary NPC and non-cancer nasopharyngeal specimens (n=96) were analysed by immunohistochemical staining with IKKα and EZH2 antibodies. Consecutive sections from three representative cases are shown. Scale bars, 100 μm. (b) Expression levels of IKKα and EZH2 were compared between undifferentiated, differentiated NPC and non-cancer group. Scores were determined as described in the Methods. (c) Model depicting the mechanism of EZH2-mediated epigenetic silencing of IKKα. In undifferentiated NPC cells, the PRC2 complex proteins EZH2 and SUZ12 are bound to theIKKα promoter where the H3K27me3 (filled circles) protein is co-occupied andIKKα transcription is suppressed. In the presence of RA, EZH2 is suppressed, which causes a reduction in H3K27 methylation (open circles). This leads toIKKα transcription that then triggers cellular differentiation. Figure 7: Low IKKα and high EZH2 correlate with undifferentiated status in NPC tissues. ( a ) Human primary NPC and non-cancer nasopharyngeal specimens ( n =96) were analysed by immunohistochemical staining with IKKα and EZH2 antibodies. Consecutive sections from three representative cases are shown. Scale bars, 100 μm. ( b ) Expression levels of IKKα and EZH2 were compared between undifferentiated, differentiated NPC and non-cancer group. Scores were determined as described in the Methods. ( c ) Model depicting the mechanism of EZH2-mediated epigenetic silencing of IKKα. In undifferentiated NPC cells, the PRC2 complex proteins EZH2 and SUZ12 are bound to the IKK α promoter where the H3K27me3 (filled circles) protein is co-occupied and IKK α transcription is suppressed. In the presence of RA, EZH2 is suppressed, which causes a reduction in H3K27 methylation (open circles). This leads to IKK α transcription that then triggers cellular differentiation. Full size image Table 1 Expression patterns of IKK α and EZH2 in consecutive sections from NPC and non-cancer tissues. Full size table Table 2 Correlation between IKK α and EZH2 levels in human primary NPC and non-cancer specimens. Full size table These new data provide compelling evidence to suggest the application of differentiation therapy as a therapeutic strategy for patients with NPC by revealing several novel findings: (1) a reduction of IKKα is involved in the undifferentiated status of NPC, (2) ectopic expression of IKKα in poorly differentiated NPC cells induces cellular differentiation in vitro and reduces tumorigenicity in vivo , (3) repression of IKKα by EZH2-induced H3K27 methylation within the IKK α promoter ultimately blocks cellular differentiation, (4) restoration of IKKα by RA promotes differentiation in NPC through inhibition of EZH2 and (5) IKKα negatively and EZH2 positively correlates with undifferentiated status in human primary NPC specimens. These data demonstrate a previously unknown but a critical pathway for the blockage of NPC cell differentiation, which is caused by EZH2-mediated epigenetic silencing of IKKα. These data provide a sound and rational biochemical basis to explore IKKα as a novel target for differentiation therapy in NPC. In the present study, we found that poorly differentiated CNE2, HONE1 and SUNE1 cells, exhibiting regular polygonal shape, expressed high level of CK13 and low levels of involucrin and CK8. Overexpression of IKKα and inhibition of EZH2, as well as RA treatment, resulted in fusiform morphological change, reduction in CK13 and increase in involucrin and CK8. These phenotypes were compatible with the well-differentiated NP69 and CNE1 cells. In addition, the induction of nasopharyngeal squamous metaplasia characterized as loss of CKs 7, 8 and 18, coupled with increased expression of CKs 1, 10 and 13, which is closely related to the histogenesis of NPC [30] , [31] . CK13 is also identified as a squamous metaplasia marker in other SCCs that originated from columnar epithelium [32] , [33] , [34] , [35] . Meanwhile, involucrin is a frequently referred marker for epithelial differentiation [36] , [37] . The induction of both CK8 and involucrin coupled with reduction of CK13 is therefore considered as markers indicating differentiation of NPC cells. However, the CK expression patterns are complicated in NPC [38] , [39] . Furthermore, morphological change of squamous carcinoma cells into fibroblast-like fusiform was associated with the dedifferentiation in some epithelial cell types [40] . More established differentiation markers, such as E-cadherin and vimentin, were thus measured in IKKα-overexpressed cells. A pattern of increased E-cadherin and decreased vimentin, along with the changes of CKs and involucrin, pointed to a phenotype of differentiation in the IKKα-overexpressed NPC cells. Previous studies have shown that IKKα plays an important role in epidermal differentiation in mice [10] , [12] , [14] . Deletion of IKK α results in a hyperproliferative and undifferentiated epidermis. Moreover, IKK α −/− keratinocytes do not respond to differentiation-inducing signals. Reintroduction of WT or kinase-inactive IKKα induced keratinocyte terminal differentiation and inhibited hyperproliferation both in vitro and in vivo [14] , [41] . These functions of IKKα are consistent with our findings that IKKα is a pivotal differentiation regulator in NPC, and overexpression of IKKα can reverse the poorly differentiated state of NPC cells by reducing proliferation and inducing differentiation. More importantly, re-expression of IKKα also reduces the tumorigenicity of NPC cells in vivo . In the present study, we found that overexpression of IKKα in the poorly differentiated CNE2 cell line resulted in a higher ability to reduce the tumorigenicity compared with knockdown of EZH2 or RA treatment. We reasoned that this finding is probably due to the reason that IKKα is the critical downstream effector activating differentiation process. Either EZH2 inhibition or RA stimulation was among the important upstream regulators to induce IKKα expression and subsequent differentiation. Moreover, using MSP analysis, the CpG islands of IKK α gene were heavily methylated in NPC cell lines and clinical specimens, compared with those in the non-cancer nasopharyngeal cell line and tissues. These results were consistent with the recent opinion that DNA methylation and histone modification cooperate to achieve silencing of target genes [26] . Thus, these results suggested that IKKα plays a key role in inducing differentiation and reducing tumorigenicity of NPC cells. The mechanism for the regulation of IKKα is not yet clearly understood, especially during tumorigenesis. MicroRNAs have been reported to be the negative regulators for IKKα. MiR-223, miR-15a, miR-16 and miR-23b reduce transcription of IKKα during macrophage differentiation and interleukin-17-associated autoimmune inflammation [42] , [43] . The p63 transcription factor, which functions as a tumour suppressor, has been found to induce IKKα expression in epithelial development and primary keratinocytes directly or indirectly [44] , [45] . Here, we demonstrate a mechanism for the downregulation of IKKα, which is associated with the poor differentiation status of NPC. Recent studies demonstrate that epigenetic regulation has a crucial function in establishing and maintaining the pattern of gene expression. Polycomb group proteins epigenetically mediate transcriptional silencing, which is involved in the maintenance of embryonic and adult stem cells and is implicated in cancer development [19] . Downregulation of IKKα expression occurs in human SCCs of the skin and lung as well as the head and neck [18] , [46] , [47] , [48] , [49] . Suppression of IKKα is associated with dedifferentiation, invasion and progression of carcinoma. Here we report that suppression of EZH2 caused a significant increase in IKKα mRNA as well as protein in NPC cells. This effect was accompanied by a reduction in the level of H3K27 methylation and an increase in transactivation of the IKK α promoter. In addition, in EZH2-silenced CNE2 cells, the PRC2 complex proteins EZH2 and SUZ12, as well as H3K27me3, showed lower occupancies at the IKK α promoter. Furthermore, overexpression of an EZH2-H694A mutant, which is HMT inactive [25] , resulted in significantly increased IKKα expression. In contrast, R732K, another SET domain mutant of EZH2 that retains HMT activity [25] , resulted in similar IKKα expression as vector control. Overexpression of EZH2-WT, however, significantly decreased IKKα expression. These results establish a mechanism where reduction of IKKα in poorly differentiated CNE2 cells is a consequence of EZH2-mediated epigenetic silencing. These new findings open avenues for differentiation therapy in NPC through targeting the EZH2-IKKα axis. A recent study showed that an EZH2 T487A mutant resulted in enhancement of EZH2 HMT activity [27] . Interestingly, although overexpression of both EZH2-WT and EZH2-T487A prevented RA-induced differentiation in CNE2 cells, we did not observe significantly stronger inhibition of differentiation using EZH2-T487A, as compared with that with EZH2-WT. We reasoned that the high HMT activity of EZH2-WT was sufficient to block RA-induced demethylation within the IKKα promoter, thus retaining cells in undifferentiated status. The objective of traditional chemotherapy or radiation therapy is to directly induce cell death. In contrast, differentiation therapy attempts to reactivate endogenous differentiation programmes in cancer cells to induce tumour cellular maturation and loss of the tumour phenotypes. A majority of NPCs arise from the mucosal epithelium of the nasopharynx, which makes surgical resection a challenging operation. Radiotherapy is the main treatment for this type of cancer, but radiotherapy often induces many undesirable side effects. NPC is a unique type of carcinoma because more than 95% of the NPCs in Southern China are undifferentiated. This unique characteristic makes NPCs an excellent model to define mechanisms for differentiation therapy. Several earlier studies showed that RA inhibits NPC cell growth, but the underlying mechanisms are not well understood [50] , [51] . Here, we used RA as a well-accepted and canonical differentiation therapy agent to demonstrate that it has the capability to induce NPC cell differentiation. It does so by abrogating EZH2-mediated epigenetic repression of IKKα. Although additional experiments will be required to further assess the therapeutic efficacy of RA in NPC patients, our data provide important implications for exploring a novel strategy of differentiation therapy in NPC. In earlier studies, RA has been reported to act via RAR/RXR signalling [52] , [53] . More recently, RA has also been showed to be involved in epigenetic regulation. For example, in primary blasts from leukaemia patients, PML-RARα recruits PRC2 and DNMTs to specific target genes, an effect that is reversed by RA treatment [54] . In accordance with these data, here we report that the binding of EZH2, SUZ12 and H3K27me3 to the IKK α promoter DNA is reduced significantly following RA treatment. In addition, RA decreased EZH2 protein in NPC cells. The specific mechanism for RA-reduced EZH2 expression in NPC cells remains to be investigated. One recent study showed that miR-214 downregulated EZH2 by targeting the EZH2 3′UTR during RA-induced differentiation in pluripotent embryonic stem cells [55] . Although miR-26a, miR-101 and miR-98 have been suggested to be involved in EZH2 regulation in NPC [56] , the mechanism remains poorly defined. Future work should address whether RA-mediated EZH2 suppression is associated with microRNA regulation. In summary, poor differentiation is a hallmark of solid tumours and is strongly related with uncontrolled growth of tumours and poor prognosis of patients. In this study, we have demonstrated that IKKα plays a pivotal and essential role in NPC differentiation and that EZH2-mediated repression of IKKα is a novel epigenetic regulatory mechanism for IKKα reduction in NPC. These data suggest a promising molecular mechanism for treatment of solid tumours and greatly strengthens the case for differentiation therapy in cancer treatment. Cell lines and culture conditions The NP69 cell line was obtained from professor Wenlin Huang (Sun Yat-sen University, Guangzhou, China). CNE1, CNE2, HK-1, HONE1 and SUNE1 cell lines were obtained from Dr Chaonan Qian (Sun Yat-sen University, Guangzhou, China). The immortalized normal human nasopharyngeal epithelial cell line NP69 was maintained in keratinocyte/serum-free medium (Invitrogen). The NPC cell lines CNE1, CNE2, HK-1, HONE1 and SUNE1 were maintained in RPMI 1640 (Invitrogen) supplemented with 10% fetal bovine serum (Hyclone). The cells were incubated at 37 °C in a humidified chamber containing 5% CO 2 . Plasmid constructs and transfection The plasmids encoding human EZH2 (wild type, WT) and human IKKα were generated by PCR amplification and subcloned into the pBabe-puro expression vector (Invitrogen). EZH2 mutant constructs EZH2 (H694A), EZH2 (R732K) were developed using the QuickChange Site directed mutagenesis kit (Stratagene) according to the manufacturer’s instructions. The mutations were chosen based on a previously published study [25] . The plasmids pCDNA-EZH2 (WT) and pCDNA-EZH2 (T487A) were provided by Mien-Chie Hung (University of Texas M.D. Anderson Cancer Center, Houston, Texas, USA) [27] , [28] . Expression plasmids were transfected into cells using Lipofectamine 2000 (Invitrogen) according to the manufacturer’s instructions. The primers for gene cloning were as follows (Invitrogen): IKKα-F 5′-ATTTGAATTCGCCACCATGGAGCGGCCCCCGGGGC-3′, IKKα-R 5′-ACGCGTCGACTCATTCTGTTAACCAACTCC-3′, EZH2-WT-F 5′-AAGGATCCATGGGCCAGACTGGGAAGA-3′, EZH2-WT-R 5′-GAGTCGACTCAAGGGATTTCCATTTCTC-3′, EZH2-H694A-F 5′-CAAAATTCGTTTTGCAAATGCTTCGGTAAATCCAAACTGC-3′, EZH2-H694A-R 5′-GCAGTTTGGATTTACCGAAGCATTTGCAAAACGAATTTTG-3′, EZH2-R732K-F 5′-CGAAGAGCTGTTTTTTGATTACAAGTACAGCCAGGCTGATGCCC-3′, EZH2-R732K-R 5′-GGGCATCAGCCTGGCTGTACTTGTAATCAAAAAACAGCTCTTCG-3′. Gene knockdown by short-hairpin RNA Knockdown of genes was performed with the specific shRNAs delivered by a lentiviral system purchased from Sigma-Aldrich Corp. according to the instruction manual. In brief, to generate the lentivirus containing specific shRNA, 293T cells were co-transfected with 2.5 μg pMD2.G and 7.5 μg psPAX2 compatible packaging plasmids and 10 μg of pLKO.1 plasmid bearing the specific shRNA for 24 h. The cultured medium containing lentivirus was collected and stored at −80 °C as aliquots for further use. To deliver the specific shRNA construct, approximately 10% confluent cells were infected with the lentivirus bearing specific shRNA in growth medium containing 8 μg ml −1 polybrene and incubated at 37 °C for 24 h. Afterwards, cells were subcultured and selected with 2 μg ml −1 puromycin. The shRNA constructs targeting the interested gene and referring to the sequence is: EZH2 (NM_004456.3): TRCN0000040074 (Insert Sequence: 5′-CCGGGCTAGGTTAATTGGGACCAAACTCGAGTTTGGTCCCAATTAACCTAGCTTTTTG-3′). The MISSION Non-Target shRNA control vector SHC002 (Insert Sequence: 5′-CCGGCAACAAGATGAAGAGCACCAACTCGAGTTGGTGCTCTTCATCTTGTTGTTTTT-3′) that contains a shRNA insert that does not target human or mouse genes was used as a negative control. Antibodies The following antibodies were used: involucrin (abcam ab14505), CK8, CK13, vimentin, IκBα and p65 (Epitomics 2032-1, 2713-1, 2707-1, 1130-1 and 1546-1, respectively), GAPDH and β-actin (proteintech 60004-1-Ig and 60008-1-Ig), IKKα (Santa Cruz sc-7218), cyclin D1, cyclin E, EZH2 and Ki67 (BD 554181, 551160, 612666 and 610969, respectively), H3K27me3 (Millipore 07-449), Histone H3, E-cadherin and SUZ12 (Cell Signaling Technology 4499, 3195 and 3737), Horseradish peroxidase-conjugated goat anti-mouse and goat anti-rabbit IgG (Pierce, 31430 and 31460), Alexa-488 and Alexa-546 (Invitrogen Molecular Probes, A11008 and A10036). Real-time RT–PCR Total RNA was extracted by using TRIzol reagent (Invitrogen), which was used to generate cDNA by using SuperScript III RT (Invitrogen) with an oligo-dT primer. Real-time RT-PCR was performed using Platinum SYBR Green qPCR SuperMix (Invitrogen) as recommended by the manufacturer. The primers used are listed in Supplementary Table 3 . GAPDH was used as the internal control. Small interfering RNA transfection RNA oligonucleotides duplexes to target genes were synthesized. Cells were seeded onto six-well plates at 16 h before transfection. In each well, 50 nM or 100 nM of siRNA and 5 μl of Lipofectamine 2000 were added to Opti-MEM, mixed and then added to the cells. After transfection of siRNAs for 24 or 48 h, RNAi efficiency was determined by real-time RT-PCR and western blot. The siRNAs were purchased from GenePharma company and the sequences were as follows: si-EZH2-1 5′-AAGAGGTTCAGACGAGCTGAT-3′, si-EZH2-2 5′-AAGACTCTGAATGCAGTTGCT-3′, si-IKKα-1 5′-GCAGGCUCUUUCAGGGACATT-3′, si-IKKα-2 5′-CAAAGAAGCUGACAAUACU-3′. Immunofluorescence staining Cells were fixed in 2% paraformaldehyde at room temperature for 20 min and permeabilized in 0.5% Triton X-100 in PBS for 10 min. Slides were incubated with the primary antibody for 60 min. The following antibodies were used: E-cadherin (1:200 dilution), vimentin (1:500 dilution), Ki67 (1:200 dilution) and p65 (1:500 dilution). Immune complexes were stained with the secondary antibody conjugated to Alexa-488 or Alexa-546 (Molecular Probes, Invitrogen, 1:200 dilution). Nuclei were stained with DAPI (Sigma-Aldrich) and viewed with an Olympus IX71 microscope. SA-β-Gal staining Cultured cells were washed in PBS and SA-β-Gal activity was detected using senescence β-gal staining kit (Sigma-Aldrich) according to the manufacturer’s directions. Air – liquid interface 3D cultured assay Cells were plated on top of a Matrigel gel containing fibroblasts (HLF cells, ATCC). After 3 days, cells were exposed to air and fed only through bottom surface, which remained in contact with the culture medium. After 14–21 days of culture, gels were fixed in formalin, embedded into paraffin, sectioned and subjected to immunohistochemical staining. The following antibodies were used: involucrin (1:200 dilution), CK13 (1:800 dilution) and vimentin (1:500 dilution). Cell cycle analysis Single-cell suspensions were fixed in ice-cold 70% ethanol for 30 min, labelled with 500 μl propidium iodide (50 μg ml −1 , Sigma-Aldrich) for at least 15 min in the dark at 37 °C and analysed directly on a Beckon Dickinson FACScan flow cytometer (Oxford, UK). Colony formation assay Approximately 500–1,000 cells were seeded into six-well plates in triplicate and incubated for 10–14 days. Colonies were stained with crystal violet and counted. Cell lysis and western blot analysis Cells were lysed on ice in RIPA buffer. Protein concentration was determined by using the Bradford dye method. Equal amounts of cell extracts were subjected to electrophoresis in 10–15% gradient SDS-PAGE gels and then transferred to nitrocellulose membranes (Millipore) for antibody blotting. The following antibodies were used: involucrin (1:1,000 dilution), CK8 (1:10,000 dilution), CK13 (1:5,000 dilution), GAPDH (1:5,000 dilution), IKKα (1:500 dilution), E-cadherin (1:1,000 dilution), vimentin (1:2,000 dilution), Cyclin D1 (1:1,000 dilution), Cyclin E (1:1,000 dilution), IκBα (1:10,000 dilution), EZH2 (1:2,000 dilution), H3K27me3 (1:1,000 dilution), Histone H3 (1:2,000 dilution) and β-actin (1:5,000 dilution). Horseradish peroxidase-conjugated goat anti-mouse or goat anti-rabbit IgG (Pierce, 1:5,000 dilution) was used as a secondary antibody. Proteins were visualized with a Super Signal West Pico chemiluminescence kit (Pierce). Uncropped scans of the most important blots used in the manuscript were shown in Supplementary Fig. 10 . Chromatin Immunoprecipitation CHIP assays were performed according to the manufacturer’s protocol (EZ-Magna ChIP kit, Millipore). Antibodies used for CHIP assay included EZH2, SUZ12 (Cell Signaling Technology) and H3K27me3 (Millipore). For sequential CHIP (Re-CHIP), the first elute immunoprecipitated by anti-EZH2 was further immunoprecipitated by anti-H3K27me3 and IgG antibodies. The percentage of bound DNA was quantified against the original DNA input. The primers used for the amplification of the precipitated DNA fragments were (position: −289/−176 within IKK α promoter): 5′-AATACAGGAGAGACTGGGCTGCTTT-3′ and 5′-GGGAGGGCTGAACGGAACCACAATG-3′. Immunohistochemical staining and statistical analysis The paraffin-embedded tissue blocks were sectioned for immunohistochemical staining [57] . Paraffin-embedded tissue specimens were sectioned, deparaffinized in xylene and rehydrated. Antigenic retrieval was processed with sodium citrate. The sections were then incubated in H 2 O 2 (3%) for 10 min, blocked in 1% bovine serum albumin for 60 min and incubated with an anti-EZH2 antibody (1:400 dilution) and anti-IKKα antibody (1:100 dilution) at 4 °C overnight. After incubation with the secondary antibody for 60 min, specimens were incubated with H 2 O 2 -diaminobenzidine until the desired stain intensity was developed. Sections were then counterstained with haematoxylin, dehydrated and mounted. Staining intensity and extent of EZH2 and IKKα expression were graded as follows: negative (score 0), bordering (score 1), weak (score 2), moderate (score 3) and strong (score 4). Extent of staining was also grouped into quintiles according to the percentage of high-staining cells in the field: negative (score 0), ⩽ 25% (score 1), 26–50% (score 2), 51–75% (score 3) and 76–100% (score 4). All immunohistochemical staining was evaluated and scored by at least two independent pathologists. Luciferase reporter assay Cells were plated at a density of 1 × 10 5 /well in 24-well plates. After 24 h, cells were transfected with IKK α promoter-driven luciferase constructs (pGL3-IKKα, kindly provide by Professor Melino G, [45] ) or control (pGL3-Basic) luciferase constructs using Lipofectamine 2000 according to the manufacturer’s instruction. Twenty-four hours after transfection, cells were harvested. Firefly and Renilla luciferase activities were measured using a dual luciferase kit (Promega). The firefly luciferase data for each sample were normalized based on transfection efficiency as measured by Renilla luciferase activity. Mouse xenograft assay Four- to six-week-old BALB/c athymic nude mice (nu/nu, male and female) were used with each experimental group consisting of 5–9 mice. In brief, mice were subcutaneously injected with cells (3 × 10 5 ~2 × 10 7 /mouse). For assay using RA, 10 days after injection, the RA group received RA (20 mg kg −1 (2d) −1 ) and the control group received equal volume of water. Tumours were measured perpendicular dimensions using calipers. Volumes were estimated using the formula ( α 2 × β )/2, where α is the shorter of the two dimensions and β is the longer one [58] . The P- value is a comparison between the control and treatment groups at the final time point when the tumours were removed from the mice. Care of experimental animals was approved by Institutional Animal Care and Use Committee of Sun-Yat-Sen University and in accordance with national guidelines for the care and maintenance of laboratory animals. Tissue samples All clinical specimens used for RNA-Seq, real-time PCR, western blot and immunohistochemical analysis were collected from NPC patients at Sun Yat-sen University Cancer Center. Patients’ consent and approval from Sun Yat-sen University Cancer Center Institute Research Ethics Committee were obtained for the use of these clinical materials. RNA-seq and accession number RNA-Seq, data generation and normalization were performed on the Illumina Cluster Station and Illumina HiSeq 2000 System at BGI and Guangzhou Genedenovo Corp. The RNA-seq data described herein have been deposited in the National Center for Biotechnology Information Sequence Read Archive ( http://www.ncbi.nlm.nih.gov/sra/ ) under accession no. SRA064011 . Methylation-specific PCR Bisulphite DNA modification was performed according to the manufacturer’s instructions (Active Motif). Primer sequences of human IKKα for the unmethylated reaction were 5′-GGAGGATTATTTGAGATTAGGAGTTT-3′ (sense) and 5′-TAAAATACAATAACACAATCACAAC-3′ (antisense) and for the methylated reaction were 5′-GGATTATTTGAGATTAGGAGTTCG-3′ (sense) and 5′-TAAAATACAATAACACGATCACGAC-3′ (antisense). Statistical analysis Each experiment was performed in triplicate and repeated at least three times. Unless otherwise indicated, data were presented as mean±s.d. of three independent experiments. Statistics were calculated by SPSS software (version 16.0). Differences among variables were assessed by two-tailed Student’s t -tests, Fisher's exact test or Pearson’s χ 2 -test. A P -value less than 0.05 was considered statistically significant (* P <0.05, ** P <0.01, *** P <0.001). How to cite this article: Yan, M. et al . IKKα Restoration via EZH2 suppression induces nasopharyngeal carcinoma differentiation. Nat. Commun. 5:3661 doi: 10.1038/ncomms4661 (2014). Accession codes: The RNA-seq data have been deposited in the NCBI Sequence Read Archive ( http://www.ncbi.nlm.nih.gov/sra/ ) under accession code SRA064011 .